Decreased CALM expression reduces Aβ42 to total Aβ ratio through clathrin-mediated endocytosis of γ-secretase A body of evidence suggests that aberrant metabolism of amyloid-β peptide (Aβ) underlies the aetiology of Alzheimer disease (AD). Recently, a single-nucleotide polymorphism in phosphatidylinositol binding clathrin assembly protein ( PICALM/CALM ) gene, which encodes a protein implicated in the clathrin-mediated endocytosis, was identified as a genetic protective factor for AD, although its mechanistic details have little been explored. Here we show that loss of CALM leads to the selective decrease in the production ratio of the pathogenic Aβ species, Aβ42. Active form of γ-secretase is constitutively endocytosed via the clathrin-mediated pathway in a CALM dependent manner. Alteration in the rate of clathrin-mediated endocytosis of γ-secretase causes a shift in its steady-state localization, which consequently impacts on the production ratio of Aβ42. Our study identifies CALM as an endogenous modulator of γ-secretase activity by regulating its endocytosis and also as an excellent target for Aβ42-lowering AD therapeutics. Amyloid-β peptide (Aβ) deposited in the brains of patients with Alzheimer disease (AD) is derived from amyloid-β precursor protein (APP) through sequential proteolytic cleavages by BACE1 and γ-secretase [1] . Cleavage of APP by γ-secretase occurs at multiple sites within the transmembrane domain to generate Aβ species with a carboxyl-terminal heterogeneity [2] , [3] . Two major forms of Aβ have distinct C termini ending at the 40th and 42nd residues (Aβ40 and Aβ42, respectively). Aβ42 is the most aggregable and massively deposited species in the brains of patients with AD and Down’s syndrome [4] . Mutations linked to familial AD (FAD) have been identified in genes encoding APP as well as presenilin (PSEN, hereafter referred to as PS), the latter being the catalytic subunit of the γ-secretase complex [5] . Previous studies revealed that several FAD mutations lead to an increased proportion of Aβ42, strongly implicating Aβ42 in the pathogenesis of AD. However, it still remains unclear whether the Aβ42 production is altered in sporadic AD as well as in ageing. Also, the regulatory mechanism that determines the γ-cleavage site remains elusive. γ-Secretase is a multimeric membrane protein complex composed of PS, nicastrin (Nct), Aph-1 and Pen-2 (refs 3 , 6 ). γ-Secretase activity is suggested to be broadly distributed between the trans -Golgi network and cell surface [7] , [8] . But recent studies including fly genetics regarding Notch processing revealed the prevalence of γ-secretase activity in late endosomes/multivesicular bodies (MVB) and lysosomes [9] , [10] . Thus, endocytic trafficking of γ-secretase might play an important role for Aβ generation, while its precise subcellular localization as well as the molecular details of the trafficking machinery of the endogenous γ-secretase still remains mostly unclear. PICALM gene has been identified as one of the genetic risk/protective factors for AD by the genome-wide association studies in late-onset AD patients [11] . Large meta-analysis of 74,046 individuals [12] revealed that carriers with minor allele (A) of rs10792832 near PICALM gene showed a decreased risk for AD with an odds ratio of 0.85–0.89. PICALM encodes a protein called CALM ( C lathrin A ssembly L ymphoid M yeloid leukemia [13] ), which has a phosphatidylinositol 4,5-biphosphate (PtdIns(4,5)P 2 ) binding ANTH domain at its N terminus, along with AP-2/clathrin binding motifs in the C-terminal region, indicating that CALM functions in the initial step of clathrin-mediated endocytosis by facilitating the proper formation of clathrin-coated pits [14] , [15] . More recently, CALM has been shown to interact directly with some of the endosomal R-SNARE proteins (that is, VAMP2, VAMP3 and VAMP8) via its ANTH domain and regulate their clathrin-dependent endocytosis [16] , suggesting its additional role in the direct recognition of endocytic cargo proteins. With regard to the relationship between CALM and the aetiology of AD, some genome-wide association studies have shown a genetic interaction of PICALM with ApoE , implying a possible involvement of CALM in the process of Aβ production/deposition [17] . Using yeast genetics and AD model mice, CALM has recently been implicated in the endocytosis of secreted Aβ and APP; however, its mechanistic details were mostly unknown [18] , [19] . Here we find that CALM regulates the endocytosis and subcellular localization of the γ-secretase and impacts on the production ratio of Aβ42. Our data raise the possibility that CALM is an endogenous γ-secretase modulator and that its variant affects the onset of AD by altering the Aβ42 production ratio in an opposite manner to that by FAD-linked mutations in APP and PS genes. Expression level of CALM is correlated with Aβ42 ratio To analyse the effect of CALM on Aβ metabolism in vivo , we measured Aβ levels in the brains of Picalm -mutant mice [20] . Previous studies have shown that changes in endogenous murine brain Aβ by overexpression/knock-in of FAD mutant PS1 (refs 21 , 22 , 23 ), or knockout of PS1 (ref. 24) [24] or BACE1 (refs 25 , 26 ) occurred in a similar manner to those observed in congenic mice crossed with human APP transgenic mice. As homozygous knockout mice show significant growth defect and die shortly after birth, we opted to use heterozygous Picalm +/− mice, which are viable with no obvious defect. Strikingly, we found that the Aβ42/total Aβ ratio, that is, proportion of Aβ42 to total Aβ (=Aβ40+Aβ42), in the soluble fraction of brain lysate of Picalm +/− mice was significantly decreased by ~20% compared with that of wild-type mice ( Fig. 1a,b ). Notably, that protein expression levels of the γ-secretase components (Nct and C-terminal fragment (CTF) of PS1) in the brains of Picalm +/− mice were increased ( Fig. 1c–e ). To investigate whether CALM affects the generation process of Aβ42, we measured Aβ secreted from cultured cells in the medium. In good agreement with the result from mouse brains, RNAi against Picalm in Neuro2a (N2a) cells, which caused near-complete depletion of CALM protein, resulted in a statistically significant reduction in Aβ42/total Aβ ratio in the secreted Aβ ( Fig. 2a–e ) regardless of the siRNA sequences ( Fig. 2d ) or APP species ( Fig. 2e ), suggesting that CALM expression levels had an impact on Aβ42 production ratio. In addition, we observed the accumulation of APP full-length (fl) protein and CTF, although APP levels were almost comparable in brains of wild-type and Picalm +/− mice (see Fig. 1 ). Next we examined the effects of overexpression of CALM in N2a cells. Alternative splicing of CALM mRNA with an internal deletion of 50 amino-acid residues was reported previously (CALM-S) [13] , [14] , although the large isoform of CALM (CALM-L) was expressed as the major species in N2a cells. However, overexpression of neither CALM-L nor CALM-S in N2a cells affected the Aβ production, supporting the notion that the formation of CALM protein complex in concert with AP-2 and clathrin heavy chain is required for the regulation of clathrin-mediated endocytosis [14] , [15] ( Fig. 2f–h ). As Aβ generation is a multi-step process, it is critical to determine which step in the Aβ generation is affected by CALM depletion. The enzymatic activity of BACE1 in the Picalm +/− brain was almost comparable to that in wild-type mice ( Fig. 3a ). We then measured Aβ secretion from CALM-depleted HeLa cells expressing APP C99, a direct γ-secretase substrate [27] . A decrease in Aβ42/total Aβ ratio was also observed ( Fig. 3b–d ), suggesting that the loss of CALM affects γ-secretase-mediated APP processing. These data suggest that the cellular amount of CALM protein correlates with the ratio of Aβ42 production at the level of γ-secretase cleavage. 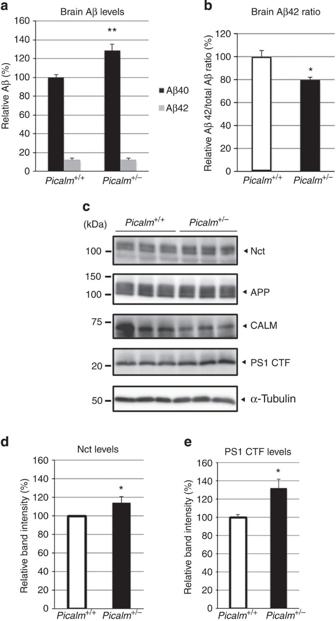Figure 1: Brain Aβ42 ratio is reduced in thePicalm+/−mouse brain. (a) Relative levels of Aβ40 and Aβ42 in Tris-soluble fraction of brains from 5-month-oldPicalm+/−or wild-type mice were quantitated by sandwich ELISAs (n=7, mean±s.e.m. **P<0.005 by student’st-test). (b) Relative Aβ42/total Aβ ratio in experiment (a) (n=7, mean±s.e.m., *P<0.05 by Student’st-test). (c) Western blot analysis of Tris-soluble fraction of brains from 5-month-oldPicalm+/−or wild-type mice with antibodies against Nct, APP, CALM, PS1 CTF and α-tubulin. Full size blots can be found inSupplementary Fig. 1. (d,e) Quantification of band intensities of total Nct (d) and PS1 CTF (e) in (c) (n=3, mean±s.e.m., *P<0.05 by Student’st-test). Figure 1: Brain Aβ42 ratio is reduced in the Picalm +/− mouse brain. ( a ) Relative levels of Aβ40 and Aβ42 in Tris-soluble fraction of brains from 5-month-old Picalm +/− or wild-type mice were quantitated by sandwich ELISAs ( n =7, mean±s.e.m. ** P <0.005 by student’s t -test). ( b ) Relative Aβ42/total Aβ ratio in experiment ( a ) ( n =7, mean±s.e.m., * P <0.05 by Student’s t -test). ( c ) Western blot analysis of Tris-soluble fraction of brains from 5-month-old Picalm +/− or wild-type mice with antibodies against Nct, APP, CALM, PS1 CTF and α-tubulin. Full size blots can be found in Supplementary Fig. 1 . ( d , e ) Quantification of band intensities of total Nct ( d ) and PS1 CTF ( e ) in ( c ) ( n =3, mean±s.e.m., * P <0.05 by Student’s t -test). 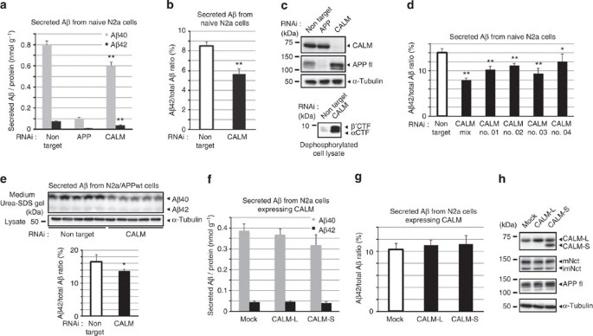Figure 2: Knockdown of CALM reduced Aβ42 ratio in secreted Aβ. (a) Levels of Aβ40 and Aβ42 secreted from N2a cells treated with non-target, APP or CALM siRNA duplex (n=6, mean±s.e.m., **P<0.005 by Student’st-test). (b) Aβ42/total Aβ ratio in experiment (a) (n=6, mean±s.e.m., **P<0.005 by Student’st-test). (c) N2a cells treated with siRNA duplexes were analysed by western blotting with antibodies against CALM, APP and α-tubulin. (d) Aβ42/total Aβ ratio in secreted Aβ in conditioned medium from N2a cells transfected with siRNAs against CALM with different target sequences. (e) Western blot analysis of the conditioned media and lysates from N2a cells stably expressing human APP by antibodies against human Aβ and α-tubulin antibody, respectively (Top panel). Aβ42/total Aβ ratio was calculated in bottom panel (n=6, mean±s.e.m., *P<0.05 by student’st-test). (f) Levels of Aβ40 and Aβ42 secreted from N2a cells transiently expressed with CALM-L or S (n=6, mean±s.e.m). (g) Aβ42/total Aβ ratio in experiment (f) (n=6, mean±s.e.m., **P<0.005 by Student’st-test). (h) N2a cell lysates in experiment (f) were analysed by western blotting with antibodies against CALM, Nct, APP and α-tubulin (mNct, mature Nct; imNct, immature Nct). Full size blots for (c), (e) and (h) can be found inSupplementary Fig. 1. Full size image Figure 2: Knockdown of CALM reduced Aβ42 ratio in secreted Aβ. ( a ) Levels of Aβ40 and Aβ42 secreted from N2a cells treated with non-target, APP or CALM siRNA duplex ( n =6, mean±s.e.m., ** P <0.005 by Student’s t -test). ( b ) Aβ42/total Aβ ratio in experiment ( a ) ( n =6, mean±s.e.m., ** P <0.005 by Student’s t -test). ( c ) N2a cells treated with siRNA duplexes were analysed by western blotting with antibodies against CALM, APP and α-tubulin. ( d ) Aβ42/total Aβ ratio in secreted Aβ in conditioned medium from N2a cells transfected with siRNAs against CALM with different target sequences. ( e ) Western blot analysis of the conditioned media and lysates from N2a cells stably expressing human APP by antibodies against human Aβ and α-tubulin antibody, respectively (Top panel). Aβ42/total Aβ ratio was calculated in bottom panel ( n =6, mean±s.e.m., * P <0.05 by student’s t -test). ( f ) Levels of Aβ40 and Aβ42 secreted from N2a cells transiently expressed with CALM-L or S ( n =6, mean±s.e.m). ( g ) Aβ42/total Aβ ratio in experiment ( f ) ( n =6, mean±s.e.m., ** P <0.005 by Student’s t -test). ( h ) N2a cell lysates in experiment ( f ) were analysed by western blotting with antibodies against CALM, Nct, APP and α-tubulin (mNct, mature Nct; imNct, immature Nct). Full size blots for ( c ), ( e ) and ( h ) can be found in Supplementary Fig. 1 . 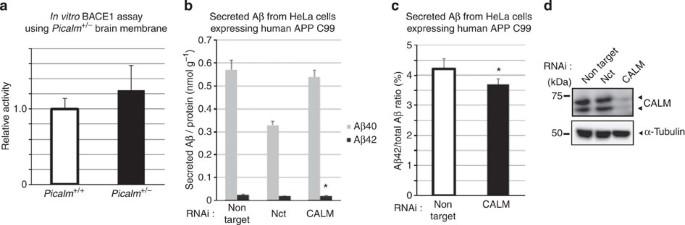Figure 3: CALM modulates the γ-secretase cleavage. (a) Relative BACE1 activity in the membrane fractions of wild-type orPicalm+/−mice brains. FRET-based BACE1 synthetic substrate was incubated with membrane fraction for 6 h, and then the fluorescence was measured (n=3, mean±s.e.m). (b) Levels of Aβ40 and Aβ42 secreted from HeLa cells expressing APP C99 treated with non-target, Nct or CALM siRNA duplexes (n=6, mean±s.e.m., *P<0.05 by Student’st-test). (c) Aβ42/total Aβ ratio in experiment (b) (n=6, mean±s.e.m., *P<0.05 by Student’st-test). (d) HeLa cells treated with non-target, Nct, or CALM siRNA duplexes were analysed by western blotting with antibodies against CALM and α-tubulin. Full size blots can be found in theSupplementary Fig. 1. Full size image Figure 3: CALM modulates the γ-secretase cleavage. ( a ) Relative BACE1 activity in the membrane fractions of wild-type or Picalm +/− mice brains. FRET-based BACE1 synthetic substrate was incubated with membrane fraction for 6 h, and then the fluorescence was measured ( n =3, mean±s.e.m). ( b ) Levels of Aβ40 and Aβ42 secreted from HeLa cells expressing APP C99 treated with non-target, Nct or CALM siRNA duplexes ( n =6, mean±s.e.m., * P <0.05 by Student’s t -test). ( c ) Aβ42/total Aβ ratio in experiment ( b ) ( n =6, mean±s.e.m., * P <0.05 by Student’s t -test). ( d ) HeLa cells treated with non-target, Nct, or CALM siRNA duplexes were analysed by western blotting with antibodies against CALM and α-tubulin. Full size blots can be found in the Supplementary Fig. 1 . Full size image CALM regulates the endocytosis of the γ-secretase complex The result that the level of γ-secretase components was increased in Picalm +/− mouse brains prompted us to speculate that CALM might affect the endocytosis and metabolism of γ-secretase. In fact, we found the accumulation of mature Nct in the lysate of CALM RNAi cells. Cell surface biotinylation experiment revealed that CALM knockdown significantly increased the levels of mature Nct at the cell surface ( Fig. 4 ). However, the intracellular localization and trafficking of γ-secretase have been under debate for years; earlier reports suggest that γ-secretase localizes at TGN, plasma membrane, endosomes and lysosomes [9] , [28] , [29] , [30] . Importantly, a detailed cell biological study of γ-secretase trafficking has been hampered because of the lack of an appropriate probe, which can specifically recognize an active, fully-assembled γ-secretase. Recently, we have developed a mouse monoclonal antibody A5226A against mature human Nct that is specifically incorporated in active γ-secretase [31] . Immunofluorescence analysis using this antibody with HeLa cells revealed that γ-secretase mostly colocalized with the late endosomal/lysosomal marker LAMP1, confirming some of the findings in the previous reports ( Fig. 5a ) [7] , [9] . Intriguingly, CALM depletion caused cell surface accumulation and less prominent late endosome localization of γ-secretase. In addition, anti-LAMP 1 staining became dispersed, suggesting that the loss of CALM caused disorganized late endosomes ( Fig. 5a ) by an impaired endocytosis of VAMP8 that is important for the fusion of late endosomes, as reported recently [16] . To investigate this further, we set up an A5226A uptake assay to monitor endocytosis of γ-secretase. In the control cells, γ-secretase is internalized slowly and started to accumulate in EEA1-positive early endosomes after 20 min of chase period and stayed there at 60 min of chase (asterisks, Fig. 5b ). Further chase visualized γ-secretase in EEA1-negative late endosomes at 480 min ( Fig. 5c ). Strikingly, A5226A uptake was markedly diminished in CALM-depleted cells ( Fig. 5b ). The majority of A5226A-labelled γ-secretase stayed at the cell surface even after 60 min of chase period (arrowheads, Fig. 5b ) and only a minor portion reached the EEA1-positive early endosomes. The endocytosis of γ-secretase was blocked also by treatment with Pitstop 2 (arrowheads, Fig. 5d ), a compound that binds to the terminal domain of clathrin heavy chain and perturbs clathrin-coated pit dynamics without affecting pit assembly nor the sequestration of the cargos [32] . Consistent with these results, a substantial colocalization of A5226A and CALM was detected at the cell surface of Pitstop 2-treated HeLa cells, a finding indicative of accumulation of γ-secretase in clathrin-coated pits in Pitstop 2-treated HeLa cells ( Fig. 5e ), suggesting that γ-secretase is internalized by clathrin-mediated endocytosis in a CALM-dependent manner. 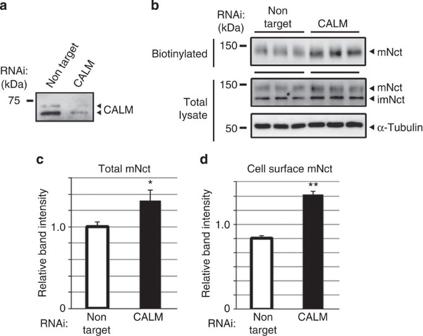Figure 4: CALM knockdown increases the expression levels of mature Nct. (a) HT1080 human fibrosarcoma cells treated with non-target or CALM were analysed by western blot. (b) Cell surface of HT1080 cells were biotinylated by NHS-SS-Biotin, and labelled proteins were selectively pulled down by streptavidin beads (mNct, mature Nct; imNct, immature Nct). (c,d) Quantification of band intensities of total mNct (c) and cell surface mNct (d) in (b) (n=3, mean±s.e.m., *P<0.05, **P<0.005 by Student’st-test). Full size blots for (a) and (b) can be found in theSupplementary Fig. 1. Figure 4: CALM knockdown increases the expression levels of mature Nct. ( a ) HT1080 human fibrosarcoma cells treated with non-target or CALM were analysed by western blot. ( b ) Cell surface of HT1080 cells were biotinylated by NHS-SS-Biotin, and labelled proteins were selectively pulled down by streptavidin beads (mNct, mature Nct; imNct, immature Nct). ( c , d ) Quantification of band intensities of total mNct ( c ) and cell surface mNct ( d ) in ( b ) ( n =3, mean±s.e.m., * P <0.05, ** P <0.005 by Student’s t -test). Full size blots for ( a ) and ( b ) can be found in the Supplementary Fig. 1 . 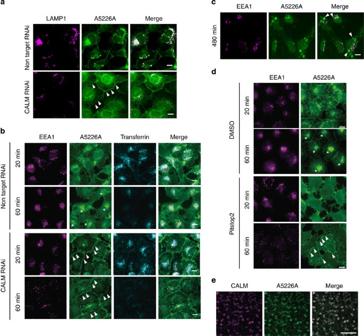Figure 5: CALM regulates clathrin-mediated endocytosis of γ-secretase. (a) HT1080 cells treated with non-target or CALM siRNA duplexes were fixed and stained with the late endosomal marker anti-LAMP1 (magenta) and anti-Nct mAb A5226A for detection of endogenous γ-secretase (green). Bar, 10 μm. (b) Uptake assay using Anti-Nct mAb A5226A and Alexa647-conjugated transferrin (cyan) in HT1080 cells treated with non-target or CALM siRNA duplexes. At the times indicated on the left, cells were fixed and stained with anti-EEA1 (magenta). A5226A bound to endogenous γ-secretase (green) was visualized by an Alexa488-conjugated anti-mouse IgG secondary antibody. Colocalization of the γ-secretase at EEA1-positive compartment as well as the cell surface accumulation of the γ-secretase is depicted by asterisks and arrowheads, respectively. Bar, 10 μm. (c) After 480 min incubation in the uptake assay, HT1080 cells were fixed and stained with anti-Nct mAb A5226A (green) and anti-EEA1 (magenta). Majority of the γ-secretase were localized at non-EEA1-positive, lysosomal compartment. Bar, 10 μm. (d) Uptake assay using Anti-Nct mAb A5226A (green) in DMSO or Pitstop 2 (30 μM)-treated HeLa cells. At the times indicated on the left, cells were fixed and stained with anti-EEA1 (magenta). Colocalization of the γ-secretase at EEA1-positive compartment as well as the cell surface accumulation of the γ-secretase is depicted by asterisks and arrowheads, respectively. Bar, 10 μm. (e) HeLa cells treated with Pitstop 2 (30 μM) for 3 h were fixed and stained with anti-Nct mAb A5226A (green) and anti-CALM (magenta). Confocal image of cell surface accumulation of the γ-secretase was taken by Leica SP5 confocal microscope. Bar, 10 μm. Full size image Figure 5: CALM regulates clathrin-mediated endocytosis of γ-secretase. ( a ) HT1080 cells treated with non-target or CALM siRNA duplexes were fixed and stained with the late endosomal marker anti-LAMP1 (magenta) and anti-Nct mAb A5226A for detection of endogenous γ-secretase (green). Bar, 10 μm. ( b ) Uptake assay using Anti-Nct mAb A5226A and Alexa647-conjugated transferrin (cyan) in HT1080 cells treated with non-target or CALM siRNA duplexes. At the times indicated on the left, cells were fixed and stained with anti-EEA1 (magenta). A5226A bound to endogenous γ-secretase (green) was visualized by an Alexa488-conjugated anti-mouse IgG secondary antibody. Colocalization of the γ-secretase at EEA1-positive compartment as well as the cell surface accumulation of the γ-secretase is depicted by asterisks and arrowheads, respectively. Bar, 10 μm. ( c ) After 480 min incubation in the uptake assay, HT1080 cells were fixed and stained with anti-Nct mAb A5226A (green) and anti-EEA1 (magenta). Majority of the γ-secretase were localized at non-EEA1-positive, lysosomal compartment. Bar, 10 μm. ( d ) Uptake assay using Anti-Nct mAb A5226A (green) in DMSO or Pitstop 2 (30 μM)-treated HeLa cells. At the times indicated on the left, cells were fixed and stained with anti-EEA1 (magenta). Colocalization of the γ-secretase at EEA1-positive compartment as well as the cell surface accumulation of the γ-secretase is depicted by asterisks and arrowheads, respectively. Bar, 10 μm. ( e ) HeLa cells treated with Pitstop 2 (30 μM) for 3 h were fixed and stained with anti-Nct mAb A5226A (green) and anti-CALM (magenta). Confocal image of cell surface accumulation of the γ-secretase was taken by Leica SP5 confocal microscope. Bar, 10 μm. Full size image This finding was consistent with the biochemical data obtained by surface biotinylation-based endocytosis assay using a cleavable biotin reagent, NHS-SS-biotin. Sodium 2-mercaptoethanesulfonate (MeSNa) treatment causes the stripping of NHS-SS-biotin from the proteins at the cell surface, but not the internalized proteins ( Fig. 6a ). Using this reagent, the amounts of biotinylated proteins that are protected by internalization can be quantitated by pull down using streptavidin beads as ‘endocytosed proteins’ after appropriate chase periods [33] . The amount of internalized pool of MeSNa-labelled Nct in the control cells was significantly higher than that in CALM siRNA-treated cells ( Fig. 6b–e ). We also found that the levels of Nct in the brains of Picalm +/− mice and CALM-depleted cells were significantly higher than those in controls ( Figs 1 and 4 ), indicating that Nct is accumulated possibly as a consequence of delayed CALM-dependent endocytosis and subsequent degradation. Previous report suggested that the endocytosis of APP and Aβ production in N2a cells overexpressing human APP was affected by CALM knockdown [19] . Importantly, cell surface levels of APP is regulated not only by endocytosis, but extracellular shedding by α-secretase. However, CALM knockdown caused a very limited effect on the amount of endocytosed MeSNa-labelled APP from the cell surface of HT1080 and N2a cells even under GM6001 treatment that inhibits shedding at the cell surface ( Fig. 6c,e ). These data suggest that endocytosis of endogenous APP is not regulated by CALM and that overexpression might have caused an overflow of exogenous APP into CALM-regulated clathrin-coated pits. Supporting this notion, reduction in total Aβ secretion by Picalm RNAi from overexpressed human APP (34.4% from stable expression, 74.4% from transient expression of non-target RNAi) was greater than that from endogenous murine APP in N2a cells (26.4% of non-target RNAi) ( Fig. 6f ). Recently, it has been reported that AP-2 and CALM bind to LC3 to facilitate the clearance of APP CTF by autophagy [34] . We examined whether APP is involved in the endocytosis of the γ-secretase by knockdown of endogenous APP. We performed the A5226A incorporation assay in APP-, CALM- and APP/CALM-knockdown cells ( Fig. 7 ). Depletion of APP expression did not affect the endocytic transport of the γ-secretase. These data suggest that APP and its binding proteins are not involved in the endocytosis of γ-secretase by CALM. 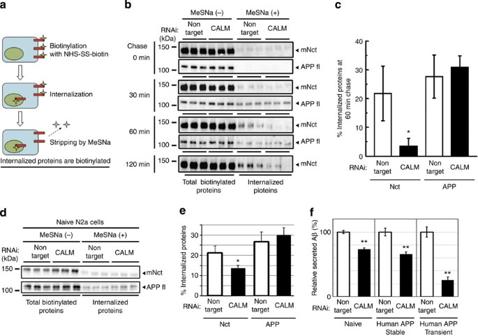Figure 6: Internalization of the γ-secretase is reduced by CALM knockdown. (a) Schematic diagram of surface biotinylation-stripping analysis to assess the rate of endocytosis using NHS-SS-Biotin. NHS-SS-biotin was cleaved by reducing reagent MeSNa to distinguish between internalized- and surface localized-proteins. (b) Effect of CALM RNAi on internalization of the γ-secretase and APP in HT1080 cells. Total biotinylated proteins (MeSNa (−)) as well as internalized proteins (MeSNa (+)) in the lysate were pulled down and visualized by western blotting. (c) Ratio of internalized proteins at 60 min chase in (b) (n=3, mean±s.e.m., *P<0.05 by Student’st-test). (d) Effect of CALM RNAi on internalization of the γ-secretase and APP in naive N2a cells at 30 min chase. (e) Ratio of internalized proteins at 60 min chase in (d) (n=3, mean±s.e.m., *P<0.05 by Student’st-test). (f) Effect of CALM RNAi on the levels of total secreted Aβ from naive, N2a cells stably or transiently expressing human APP measured by ELISA (n=6, mean±s.e.m., **P<0.005 compared with each non-target RNAi by Student’st-test). Human Aβ-specific ELISA system was used for the detection of Aβ from transfected human APP. Full size blots of (b) and (d) can be found inSupplementary Fig. 1. Figure 6: Internalization of the γ-secretase is reduced by CALM knockdown. ( a ) Schematic diagram of surface biotinylation-stripping analysis to assess the rate of endocytosis using NHS-SS-Biotin. NHS-SS-biotin was cleaved by reducing reagent MeSNa to distinguish between internalized- and surface localized-proteins. ( b ) Effect of CALM RNAi on internalization of the γ-secretase and APP in HT1080 cells. Total biotinylated proteins (MeSNa (−)) as well as internalized proteins (MeSNa (+)) in the lysate were pulled down and visualized by western blotting. ( c ) Ratio of internalized proteins at 60 min chase in ( b ) ( n =3, mean±s.e.m., * P <0.05 by Student’s t -test). ( d ) Effect of CALM RNAi on internalization of the γ-secretase and APP in naive N2a cells at 30 min chase. ( e ) Ratio of internalized proteins at 60 min chase in ( d ) ( n =3, mean±s.e.m., * P <0.05 by Student’s t -test). ( f ) Effect of CALM RNAi on the levels of total secreted Aβ from naive, N2a cells stably or transiently expressing human APP measured by ELISA ( n =6, mean±s.e.m., ** P <0.005 compared with each non-target RNAi by Student’s t -test). Human Aβ-specific ELISA system was used for the detection of Aβ from transfected human APP. Full size blots of ( b ) and ( d ) can be found in Supplementary Fig. 1 . 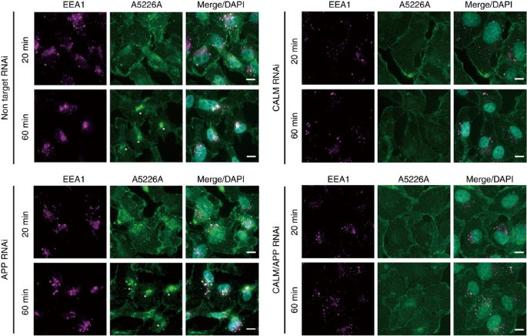Figure 7: APP knockdown unaffected the endocytosis of the γ-secretase. Uptake assay using Anti-Nct mAb A5226A in HT1080 cells treated with non-target, CALM or APP siRNA. At the times indicated on the left cells were fixed and stained with anti-EEA1 (magenta) asFig. 5. Colocalization of the γ-secretase at EEA1-positive compartment are depicted by asterisks. Bar, 10 μm. Full size image Figure 7: APP knockdown unaffected the endocytosis of the γ-secretase. Uptake assay using Anti-Nct mAb A5226A in HT1080 cells treated with non-target, CALM or APP siRNA. At the times indicated on the left cells were fixed and stained with anti-EEA1 (magenta) as Fig. 5 . Colocalization of the γ-secretase at EEA1-positive compartment are depicted by asterisks. Bar, 10 μm. Full size image CALM has been shown to regulate the endocytosis of a subset of membrane proteins as its cargo [14] , [20] , [35] , [36] , [37] . In regard to the recognition of the cargo, it has recently been shown that VAMP8, one of the R-SNARE proteins, binds directly to the C-terminal edge of ANTH domain and is internalized in a CALM-dependent manner [16] . To test the possibility that CALM also directly recognizes γ-secretase as an endocytic cargo, we carried out an in vitro binding experiment using GST-fused recombinant CALM proteins encoding an N-terminal PtdIns(4,5)P 2 binding ANTH domain or the C-terminal region, which contains multiple clathrin and AP-2 binding motifs (ΔN) ( Fig. 8a ). We confirmed that VAMP8 as well as AP-2 specifically interacted with the recombinant ANTH domain and ΔN protein of CALM, respectively ( Fig. 8b ). Unexpectedly, AP-2 also interacted with the ANTH domain, raising the possibility that this region contains a novel AP-2 binding domain. In this condition, we found that endogenous Nct also bound to the ANTH domain, but not with the ΔN protein ( Fig. 8b ). The majority of GST-ANTH bound Nct was in its immature form, which represents the Nct species residing at ER. However, this band was not present in lysates from fibroblast of Ncstn knockout mice, and detected upon transfection of human Nct-V5, indicating that this polypeptide is Nct ( Fig. 8c ). In addition, we did observe the binding of mature Nct that locates at the cell surface (see Fig. 8c–e and discussed below). As Nct initially forms a subcomplex with Aph-1 and then binds to the C terminus of PS during the assembly process of γ-secretase [6] , [7] , it is possible that Nct indirectly interacts with the ANTH domain through other subunits. However, interaction of Nct with recombinant ANTH domain was also observed in the lysates of fibroblasts lacking PS or Aph-1, indicating that CALM directly recognizes Nct as an endocytic cargo in the γ-secretase complex ( Fig. 8d ). Notably, VAMP8 knockdown caused no difference, rather, a slight increase in the amount of Nct associated with the ANTH domain, suggesting a possible competition between Nct and VAMP8 for their binding to the ANTH domain ( Fig. 8e ). Taken together, for the first time, we have shown that γ-secretase is constitutively internalized via the clathrin-dependent pathway as the endocytic cargo of CALM ( Fig. 8f ). 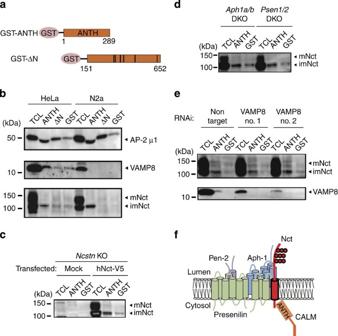Figure 8: CALM directly recognizes γ-secretase. (a) Schematic depiction of recombinant proteins used in this study. (b) GST pull-down assay using HeLa or N2a cell lysates. Bound proteins were analysed by western blotting using antibodies against AP-2, VAMP8 and Nct (mNct, mature Nct; imNct, immature Nct). (c) GST pull-down assay using lysates fromNcstnknockout fibroblast cells expressing mock or human Nct with C-terminal V5 tag. (d) GST pull-down assay using lysates fromAph1a/bDKO andPsen1/2DKO fibroblast cells. (e) Effect of VAMP8 knockdown on the interaction between CALM and Nct. Two different siRNAs were treated with HeLa cells, and GST pull-down assay was performed as in (a). (f) Schematic depiction of the binding of CALM and Nct in the γ-secretase complex. Full size blots of (b–e) can be found inSupplementary Fig. 1. Figure 8: CALM directly recognizes γ-secretase. ( a ) Schematic depiction of recombinant proteins used in this study. ( b ) GST pull-down assay using HeLa or N2a cell lysates. Bound proteins were analysed by western blotting using antibodies against AP-2, VAMP8 and Nct (mNct, mature Nct; imNct, immature Nct). ( c ) GST pull-down assay using lysates from Ncstn knockout fibroblast cells expressing mock or human Nct with C-terminal V5 tag. ( d ) GST pull-down assay using lysates from Aph1a/b DKO and Psen1/2 DKO fibroblast cells. ( e ) Effect of VAMP8 knockdown on the interaction between CALM and Nct. Two different siRNAs were treated with HeLa cells, and GST pull-down assay was performed as in ( a ). ( f ) Schematic depiction of the binding of CALM and Nct in the γ-secretase complex. Full size blots of ( b – e ) can be found in Supplementary Fig. 1 . Full size image Aβ42 production ratio is increased by acidic pH To test whether loss of CALM directly affects the enzymatic function of γ-secretase, we performed an in vitro γ-secretase assay using detergent-solubilized membrane fractions from CALM-depleted cells ( Fig. 9 ). We observed no decrease in the Aβ42/total Aβ ratio of the de novo generated Aβ, suggesting that the intrinsic enzymatic activity of γ-secretase was not affected by CALM knockdown. Then we turned our attention to the finding that the localization of γ-secretase changed upon depletion of CALM. It led us to speculate that γ-secretase activity was affected by its altered subcellular localization. To explore this possibility, we took a pharmacological approach utilizing YM201636, which inhibits the phosphatidylinositol 3-phosphate 5-kinase Pikfyve. Pikfyve phosphorylates PtdIns3P to generate PtdIns(3,5)P 2 and is responsible for the maturation of early endosomes/multivesicular bodies into the degradative late endosomes/lysosomes [38] . YM201636 treatment caused increased vacuolation and redistribution of EEA1 and LAMP1 as reported previously [38] ( Fig. 10a ). Intriguingly, YM201636 caused a reduction in the Aβ42/total Aβ ratio in the secreted Aβ as well as accumulation of mature Nct, APP full length and CTF, similarly to those in CALM-depleted cells ( Fig. 10b–d ). Consistent with this, knockdown of YM201636-target kinase Pikfyve also reduced the Aβ42/total Aβ ratio, along with accumulation of APP and CTFs ( Fig. 10e–g ), suggesting that Pikfyve-mediated late endosomal maturation is closely involved in the Aβ42 production. However, incubation of the membrane fraction from YM201636-treated cells showed no difference in Aβ42/total Aβ ratio in de novo -generated Aβ ( Fig. 10h ), suggesting that the decrease in Aβ42/total Aβ ratio by YM201636 was not caused by an altered membrane lipid composition (that is, decreased PtdIns(3,5)P 2 levels). During the endosomal maturation, the lumen of the organelle is gradually acidified as it progresses towards lysosomes. To test whether acidification of endosome is critical to Aβ42 production, we tested several different pH upon membrane incubation. Notably, Aβ42/total Aβ ratio was increased along with decreased pH ( Fig. 10i ). These data suggest that the degree of acidification in the endosomal compartment, where the γ-secretase resides, is responsible for the increases in Aβ42/total Aβ ratio in the γ-cleavage. 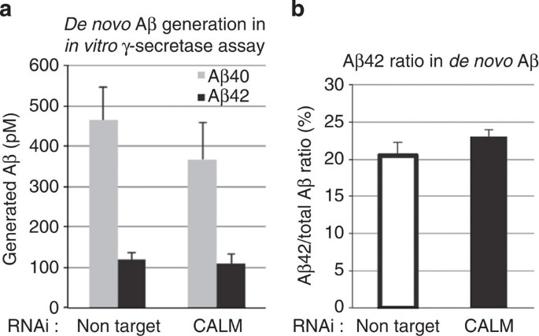Figure 9: Intrinsic enzymatic activity of the γ-secretase in CALM-depleted cell membranes. Levels ofde novoAβ generation (a) and Aβ42/total Aβ ratio (b) inin vitroγ-secretase assay using cell membrane treated with non-target or CALM siRNA duplexes (n=3, mean±s.e.m). Figure 9: Intrinsic enzymatic activity of the γ-secretase in CALM-depleted cell membranes. Levels of de novo Aβ generation ( a ) and Aβ42/total Aβ ratio ( b ) in in vitro γ-secretase assay using cell membrane treated with non-target or CALM siRNA duplexes ( n =3, mean±s.e.m). 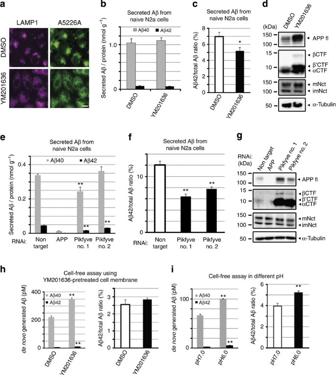Figure 10: Acidification in the consequence of endosomal maturation is the critical determinant for Aβ42 ratio. (a) Effect of YM201636 on the localization of LAMP1-positive compartment and the endogenous γ-secretase in HeLa cells. Bar, 10 μm. (b,c) Levels of secreted Aβ from N2a cells (n=3, mean±s.e.m) (b) and Aβ42/total Aβ ratio (c) treated with DMSO or YM201636 (n=3, mean±s.e.m., *P<0.05 by Student’st-test). (d) N2a cells treated with DMSO or YM201636 were analysed by western blotting with antibodies to APP, Nct and α-tubulin (mNct, mature Nct; imNct, immature Nct). (e,f) Effect of knockdown of Pikfyve on secreted Aβ levels from N2a cells (n=6, mean±s.e.m., **P<0.005 by Student’st-test) (e), Aβ42/total Aβ ratio (f) (n=6, mean±s.e.m., **P<0.005 by Student’st-test). (g) N2a cells treated with APP or Pikfyve siRNA duplexes were analysed by western blotting with antibodies to APP, Nct and α-tubulin. (h) Levels (left) and Aβ42/total Aβ ratio (right) inde novoAβ generated in cell-free assay using membranes obtained from APP695-expressing HEK293 cells pretreated with DMSO or YM201636 (n=3, mean±s.e.m., **P<0.005 by Student’st-test). (i) Levels (left) and Aβ42/total Aβ ratio (right) inde novoAβ generated in cell-free assay using APP695-expressing HEK293 cell membranes under different pH condition (7.0 or 6.0) (n=3, mean±s.e.m., **P<0.005 by Student’st-test). Full size blots for (d) and (g) can be found inSupplementary Fig. 1. Full size image Figure 10: Acidification in the consequence of endosomal maturation is the critical determinant for Aβ42 ratio. ( a ) Effect of YM201636 on the localization of LAMP1-positive compartment and the endogenous γ-secretase in HeLa cells. Bar, 10 μm. ( b , c ) Levels of secreted Aβ from N2a cells ( n =3, mean±s.e.m) ( b ) and Aβ42/total Aβ ratio ( c ) treated with DMSO or YM201636 ( n =3, mean±s.e.m., * P <0.05 by Student’s t -test). ( d ) N2a cells treated with DMSO or YM201636 were analysed by western blotting with antibodies to APP, Nct and α-tubulin (mNct, mature Nct; imNct, immature Nct). ( e , f ) Effect of knockdown of Pikfyve on secreted Aβ levels from N2a cells ( n =6, mean±s.e.m., ** P <0.005 by Student’s t -test) ( e ), Aβ42/total Aβ ratio ( f ) ( n =6, mean±s.e.m., ** P <0.005 by Student’s t -test). ( g ) N2a cells treated with APP or Pikfyve siRNA duplexes were analysed by western blotting with antibodies to APP, Nct and α-tubulin. ( h ) Levels ( left ) and Aβ42/total Aβ ratio ( right ) in de novo Aβ generated in cell-free assay using membranes obtained from APP 695 -expressing HEK293 cells pretreated with DMSO or YM201636 ( n =3, mean±s.e.m., ** P <0.005 by Student’s t -test). ( i ) Levels ( left ) and Aβ42/total Aβ ratio ( right ) in de novo Aβ generated in cell-free assay using APP 695 -expressing HEK293 cell membranes under different pH condition (7.0 or 6.0) ( n =3, mean±s.e.m., ** P <0.005 by Student’s t -test). Full size blots for ( d ) and ( g ) can be found in Supplementary Fig. 1 . Full size image Here, we provide striking evidence for the first time that γ-secretase is constitutively internalized via clathrin-mediated endocytosis, which is regulated by CALM. The precise subcellular localization of the active γ-secretase has been enigmatic for a long time [8] . Recent studies including fly genetics revealed the prevalence of Notch processing along the endolysosomal system [10] . However, the trafficking itinerary of γ-secretase, as well as the identity of its regulatory mechanism, has rarely been described. Our results presented here clearly indicate that γ-secretase is endocytosed from the cell surface and transported to lysosomes, and that this pathway is regulated by CALM. Moreover, intriguingly, binding assay revealed that CALM directly recognizes Nct as an endocytic cargo in the γ-secretase complex. Unexpectedly, significant amount of immature Nct was detected in the ANTH domain-bound fraction, whereas mature Nct was the only species that locates at the cell surface. Considering the previous report that Nct C-terminally fused with ER-retention signal was still capable of forming active γ-secretase and maturated [39] , steric hindrance of the C terminus of Nct would have occurred upon the assembly of the complex. This raises the possibility that as yet unknown signal or post-translational modifications induce a structural change in the cytoplasmic domain of Nct and allow the binding to CALM, resulting in enhanced endocytosis. We have also shown that the extents of reduction in total Aβ secretion from endogenous, stably expressed and transiently expressed APP were varied ( Fig. 6f ). Total Aβ production is correlated with β-cleavage that requires endocytosis of APP [40] . Thus, overexpressed APP might overflow into the clathrin-coated pits regulated by CALM. This might be a reason why significant reduction in Aβ secretion was observed in knockdown experiments by Xiao et al . [19] as well as the transient expression of APP ( Fig. 6f ). However, Aβ42 ratio was altered in heterozygous knockout mice brains, while total Aβ level was unchanged, suggesting that the alteration of the γ-secretase activity is more sensitive than that of APP. As to the physiological significance of this CALM-dependent γ-secretase endocytosis, it has been shown that Notch S3 processing by γ-secretase at the cell surface produces stable NICD starting at Val residue, whereas its endosomal processing produces shorter, unstable NICD leading to the attenuated signalling [41] . This implies that the magnitude of Notch signalling is controlled not only by the trafficking of Notch itself but also that of γ-secretase. Whether γ-secretase activity is regulated by membrane traffic in response to specific signalling pathways will be an important area for further investigation. Also intriguing is the finding that loss of CALM alters proteolytic activity of γ-secretase to reduce the production ratio of Aβ42, consistently observed both in vitro and in vivo . To date, several protective mutations/variants against AD have been reported by genome-wide association studies and whole-genome sequencing. Among these variants, a rare variant causing A673T substitution of APP gene reduced Aβ production by affecting β-cleavage [42] , and minor allele (A) of rs3865444 in CD33 gene regulated the phagocytosis of Aβ by microglia [43] , [44] . Considering the fact that almost all of FAD-linked mutations increase the production/aggregation of Aβ in vitro as well as in vivo , modulation of brain Aβ levels is crucial to the molecular aetiology of AD. However, no genetic variant altering the γ-secretase activity has been reported, although γ-secretase modulator has been regarded as a promising treatment [1] . Our present result suggests that the minor allele (A) of rs10792832 near PICALM gene would affect the expression of CALM in a way to reduce the production ratio of Aβ42, thereby leading to a protective effect against AD [12] . Importantly, reduced Aβ42/total Aβ ratio was recapitulated by treatment with YM201636 that blocks endosomal maturation and redistributes γ-secretase to the earlier endocytic compartment. These results suggest that the change in the steady-state localization of γ-secretase, which is determined by the balance between endolysosomal trafficking and recycling to the cell surface, is correlated with the lowered Aβ42/total Aβ ratio. Notably, in YM201636 treated cells, we did not observe changes in the total level of Aβ secretion, while incubation of membrane fractions obtained from YM201636-treated cells increased the production of Aβ. It is tempting to speculate that the endolysosomal maturation is required for not only the production but also secretion of Aβ. Nevertheless, CALM depletion appears to shift the balance towards recycling, so that γ-secretase accumulates at the earlier endocytic compartment where it preferentially cleaves APP CTF at Aβ40 position. Why does this change in localization matter? It has been shown biochemically that subcellular localization affects the proteolytic activity of γ-secretase and this might be attributed to the difference in membrane lipid composition or pH [41] , [45] , [46] . As shown in this study, low pH caused a significant increase in Aβ42/total Aβ ratio in an in vitro assay, indicating that alteration of pH along with endosomal maturation has an impact on the γ-secretase activity for Aβ42 production ratio. Our findings also raise the possibility that inhibition of CALM function as well as of endosomal maturation of γ-secretase is considered as a promising therapeutic target of AD. While total systemic loss of CALM in mice leads to neonatal death possibly due to impaired iron uptake and other crucial endocytosis, heterozygous mice showed no obvious abnormalities [20] . Reduced Aβ42/total Aβ ratio in heterozygous mouse brain suggests that partial inhibition of CALM function could be enough to prevent the development of AD with minimal side effects. In this regard, it is noteworthy to mention that Ca 2+ -dependent synaptic vesicle exocytosis has been shown to modulate PS1 conformation and the Aβ42 production ratio [47] . As CALM is essential to the endocytic pathway of synaptic vesicles [48] , CALM would be a critical regulator of neuronal activity-dependent Aβ42 production ratio. Notably, the magnitude of reduction in Aβ42 ratio by CALM knockdown varied with different APP constructs (Compare Figs 2b,e and 3c ). One possibility is that subcellular location of β-cleavage of APP, which should precede the γ-cleavage, is correlated with this difference in the reduction of Aβ42 ratio. In fact, recent studies indicate that β-cleavage of APP is dynamically regulated by membrane trafficking [49] , [50] , [51] as well as neuronal activity [40] , [52] . SNPs found in the late-onset AD patients are associated with the disease with a reduced risk, so it would be interesting to see whether the expression level or function of CALM is lowered in the brains of patients carrying these SNPs. CALM knockdown slowed, but did not abolish, the endocytosis of the γ-secretase, suggesting that other factors or molecular systems including AP180 would complement the trafficking of the γ-secretase upon depletion of CALM function within cells. In summary, we have identified CALM as a regulator of γ-secretase endocytosis and Aβ42 production ratio. This study is an important step forward in understanding the cell biology of γ-secretase as well as defining a novel target for the anti-amyloid treatment of AD. Molecular biology Human CALM (long (CALM-L) and short (CALM-S) isoforms, NCBI nucleotide accession number BC048259 and BC064357, respectively) and human BACE1 (BC065492) ORFs were amplified from IMAGE clones (Open Biosystems) using KOD plus neo DNA polymerase (TOYOBO). Expression constructs encoding wild-type human APP 695 full length and C99 were described before [27] . Mammarian expression constructs were made using pEF6-V5 His TOPO TA or pcDNA3.1-hygro vector (Invitrogen). Bacterial expression constructs for recombinant GST fusion proteins were made using pFAT2 vector encoding Hisx6-Gultathion S transferase (GST). The following ON-TARGETplus SMARTpool small interfering RNAs (Thermo Scientific) were used against human Nct (#L-008043-00), human APP (#L-003731-00), mouse APP (#L-043246-00), human CALM (#L-004004-00), mouse CALM (#L-041440-01). Luciferase GL2 (#D-001100-20) and Non-targeting pool (#D-001810-10) were used as control siRNAs. SiRNAs targeting human VAMP8 (SI 02652993 and SI04437804) were purchased from Qiagen. Antibodies and chemicals The following antibodies were purchased from commercial suppliers: anti-CALM (sc-6433, Santa Cruz, 1:1,000 dilution for western blot analyses, 1:400 dilution for immunocytochemical analysis), anti-APPc (#18961, Immuno-Biological Laboratories, 1:1,000), anti-human Aβ specific antibody 82E1 (#10323, Immuno-Biological Laboratories, 1:1,000 dilution), anti-α-tubulin DM1A (T6199, Sigma, 1:2,000 dilution), anti-Nct N terminus (sc-14369, N-19; Santa Cruz, 1:1,000 dilution), anti-Nct C terminus (N1660, Sigma, 1:1,000 dilution), anti-LAMP1 (#328611, Alexa-647 tagged antibody, Bio Legend, 1:500 dilution), anti-EEA1 (#2411S, Cell Signaling Technology, 1:200 dilution), anti-AP-2μ1 (#2386-1, Epitomics, 1:1,000 dilution), anti-VAMP8 (ab76021, Abcam, 1:5,000 dilution). Rabbit polyclonal anti-PS1 CTF antibody G1L3 and mouse monoclonal anti-Nct A5226A were described previously [31] , [53] . Pitstop 2 and YM201636 were purchased from Abcam and Cayman Chemicals, respectively. Cell culture and RNA interference HeLa S3 (#CCL-2.2, ATCC), Neuro2a (N2a) (#CCL-131, ATCC), HT1080 (provided from Dr. Masatoshi Maki (Nagoya University)), HEK293 (#CCL-1573, ATCC), embryonic fibroblast cells obtained from Ncstn −/− , Psen1 −/− ;Psen2 −/− and Aph1a −/− ;Aph1b −/− mice ( Ncstn KO, Psen1/2 DKO and Aph1a/b DKO MEFs, respectively) [54] , [55] , [56] were cultured in DMEM supplemented with 10% fetal calf serum. N2a cells stably expressing human wild-type APP 695 were selected using 50 μg ml −1 Blasticidin S (Calbiochem). Flp-In T-REx-293 cell lines stably expressing Tet-inducible human wild-type APP 695 were selected using 200 μg ml −1 Hygromycin according to the manufacturer’s protocol (Invitrogen). Ncstn KO MEF cells stably expressing V5/His-tagged Nct were selected using 10 μg ml −1 Blasticidin (Calbiochem) [57] . siRNAs were transfected into 20~30% confluent cells using LipofectAMINE RNAiMAX (Invitrogen) at a concentration of 20 nM, and cells and culture medium were analysed 48–72 h after transfection. In experiments in which a combination of siRNA and plasmid delivery was necessary, plasmids were transfected with TransIT-2020 (Mirus) or Fugene 6 (Roche Applied Science) 24 h after siRNA delivery. For immunocytochemical analysis, cells cultured on glass coverslips were fixed for 15 min in 4% paraformaldehyde and then permeabilized with 0.2% Tx-100 for 10 min. All solutions were made in PBS. Coverslips were then incubated with primary antibodies as indicated for 1 h. After washing with PBS, coverslips were incubated with secondary antibodies for 1 h and washed with PBS, mounted on slide glass using PermaFluor Aqueous Mounting Medium (Thermo Scientific) mixed with 1 μg ml −1 DAPI for nuclear staining. Images were collected with either a fluorescence microscope (AxioObserver Z1, Zeiss) with a × 40 Plan Apochromat oil immersion objective of NA 1.3, AxioVision software or a confocal microscope (SP5, Leica) with a × 63 PL APO CS oil immersion objective of NA 1.4, Leica LAS AF software. Images were cropped and processed using ImageJ software (NIH). To detect colocalization of CALM and Nct, subconfluent cells were treated with 30 μM Pitstop 2 in DMEM without FBS for 3 h before fixation. For western blot analyses, cells were lysed by Laemlli sample buffer and sonicated. Protein concentration was measured by using BCA protein assay (Pierce). For detection of APP CTFs, cell lysates (40 mg of protein) were dephosphorylated by recombinant Lambda protein phosphatase (400 unit; New England Biolabs) for 4 h at 30 °C (ref. 58 ). Secreted human Aβ was separated in Urea-SDS PAGE gel [59] and detected by western blotting using a human Aβ specific antibody 82E1. Brain extraction All experiments using animals in this study were performed according to the guidelines provided by the Institutional Animal Care Committee of Graduate School of Pharmaceutical Sciences, The University of Tokyo. All animals (5-month-old mice, female) were maintained on food and water with a 12 h light/dark cycle. The brains that were excised from 5 months old of Picalm +/− or wild-type mice were homogenized in RIPA buffer (Thermo Scientific) containing Complete protease inhibitor cocktail (Roche Applied Science). Homogenates were cleared by centrifugation at 200,000 × g for 20 min at 4 °C, and the resultant supernatant was collected as brain RIPA extract. The RIPA extract was used for quantitation of Aβ by ELISA (Human/Rat beta-Amyloid (40) ELISA Kit (#294-62501, WAKO Pure Chemical Industries) and Human/Rat β-Amyloid (42) ELISA Kit, High Sensitivity (#292-64501, WAKO Pure Chemical Industries) and also analysed by SDS-PAGE and western blots. For in vitro BACE1 assay, the RIPA extract was acidified by 25 mM CH 3 COONa pH 4.5 and incubated with the β-secretase-specific recombinant peptide-based substrate JMV2236 (Bachem) at 37 °C at the indicated times. Fluorescence of the fractions was measured at 320 and 420/430 nm as excitation and emission wavelengths, respectively [60] . Ligand uptake assays Subconfluent HeLa or HT1080 cells were incubated in the medium containing 50 μg ml −1 Alexa-647 transferrin and 10 μg ml −1 anti-Nct MAb A5226A for 20 min at 37 °C. After washing with medium, fresh prewarmed medium was added and further incubated for varying times at 37 °C. Cells were then washed immediately with PBS, fixed in PFA and processed for immunocytochemical analysis. Cell-surface biotinylation-based endocytosis assay Cell-surface biotinylation-based endocytosis assay was performed according to the method established by Bretscher and Lutter [61] with some modifications. In brief, near-confluent cells were washed with ice-cold PBS and then incubated on ice with a membrane-impermeant, cleavable biotin derivative Sulfo-NHS-SS-Biotin (Thermo Scientific, 1 mg ml −1 in PBS) for 30 min to label surface proteins. Excess biotin reagent was quenched by washing cells three times with 0.1 M glycine in PBS. Cells were rinsed with ice-cold PBS and re-fed with prewarmed and CO 2 equilibrated growth medium including 20 μM GM6001 (Calbiochem) (except for ‘t0’ sample). Cells were then incubated for varying times at 37 °C to allow internalization. At each time point, cells were transferred to ice to terminate internalization, washed with ice-cold PBS twice and then stripped of remaining surface biotin by washing three times for 20 min on ice in biotin-stripping buffer (50 mM Tris pH 8.6, 100 mM NaCl, 1 mM EDTA and 0.2% purified BSA, 100 mM sodium 2-mercaptoethanesulfonate (MeSNa)). After quenching MeSNa by incubating for 10 min on ice in PBS containing 120 mM Iodoacetic acid followed by washing with ice-cold PBS twice, cells were lysed in PBS containing 1% SDS. The lysates were then sonicated and biotinylated proteins were captured with streptavidin sepharose (GE Healthcare) for 12 h on a rotary mixer, eluted in SDS sample buffer by boiling for 1 min and analysed by western blotting. Protein expression and purification CALM ANTH domain (1–289) and ΔN protein (151–652) were expressed as His- GST-fusion proteins in Escherichia coli BL21(DE3) (WAKO). Cells were grown to mid log, induced with 0.2 mM IPTG for 2.5 h at 37 °C. Bacterial lysates were prepared from pellets by sonication in E coli lysis buffer (20 mM Tris–HCl pH8.0, 300 mM NaCl, 20 mM imidazole, 0.1% Triton X-100), cleared by centrifugation and His-GST-fusion proteins were purified on Ni-NTA agarose (Qiagen) in 20 mM Tris–HCl pH 8.0, 300 mM NaCl, 20 mM Imidazole and eluted in the same buffer but now containing 200 mM imidazole. Proteins were dialysed against Tris-buffered saline (50 mM Tris–HCl pH8.0, 150 mM NaCl) and then aliquots were frozen in liquid nitrogen for storage at −80 °C. HeLa, N2a and Ncstn KO MEF cell lysates were prepared by using mammalian cell lysis buffer (20 mM Tris–HCl, pH 7.6, 150 mM NaCl, 0.5% Triton X-100) containing Complete protease inhibitor cocktail and precleared by incubating with glutathione sepharose (GE Healthcare) for 1 h. In pull-down experiments, 1 mg of cleared total cell lysate and 200 μg of GST-CALM proteins were mixed in lysis buffer. Following the addition of 50 μl glutathione sepharose beads, the mixture was incubated for 90 min at 4 °C on a rotator. The glutathione sepharose beads were washed three times with lysis buffer. After washing, 100 μl of 2 × sample buffer was added to the beads for elution and boiled for 1 min. Bound proteins were analysed by SDS-PAGE and western blots. GST alone served as a negative control. In vitro γ-secretase assays For secreted Aβ levels, conditioned media from N2a cells, HEK293 cells stably expressing wild-type human APP 695 or HeLa cells co-expressing wild-type human APP 695 and BACE1 were analysed by two-site enzyme-linked immunosorbent assay (ELISA) [62] . For cell-free γ-secretase assay, membranes of HEK293 cells stably expressing APP were collected and analysed as described previously [63] . In all, 2.5 mg ml −1 microsomes in homogenize buffer (20 mM HEPES pH 7.0, 140 mM KCl, 250 mM sucrose, 5 mM EGTA) containing 0.5 mM DIFP, 0.5 mM PMSF, 1 μg ml −1 TLCK, 1 μg ml −1 antipain, 1 μg ml −1 leupeptin, 10 μg ml −1 phosphoramidon, 1 mM EGTA, 5 mM EDTA, 5 mM 1,10-Phenanthroline were preincubated with L-685,458 or DMSO on ice for 30 min. Microsomes were incubated at 37 °C for 6 h and then centrifuged at 15,000 rpm for 10 min. The supernatant was analysed by ELISA. In experiments in which cell-free γ-secretase assays were performed under different pH conditions, citric acid-Na 2 HPO 4 buffer was used instead of HEPES buffer. For in vitro γ-secretase assay, 1% CHAPSO-solubilized membranes from HeLa cells were incubated with APP-based recombinant substrate C100-Flag/Myc/His purified from Escherichia coli under 0.25% CHAPSO condition [6] , [64] and then analysed by ELISA. Statistical analysis Data are presented as mean values and error bars indicate s.e.m. The treatment groups were compared by two-tailed Student’s t -test. Significance was set at * P <0.05 and ** P <0.005. How to cite this article: Kanatsu, K. et al. Decreased CALM expression reduces Aβ42 to total Aβ ratio through clathrin-mediated endocytosis of γ-secretase. Nat. Commun. 5:3386 doi: 10.1038/ncomms4386 (2014).